FAD-dependent lysine-specific demethylase-1 regulates cellular energy expenditure Environmental factors such as nutritional state may act on the epigenome that consequently contributes to the metabolic adaptation of cells and the organisms. The lysine-specific demethylase-1 (LSD1) is a unique nuclear protein that utilizes flavin adenosine dinucleotide (FAD) as a cofactor. Here we show that LSD1 epigenetically regulates energy-expenditure genes in adipocytes depending on the cellular FAD availability. We find that the loss of LSD1 function, either by short interfering RNA or by selective inhibitors in adipocytes, induces a number of regulators of energy expenditure and mitochondrial metabolism such as PPARγ coactivator-1α resulting in the activation of mitochondrial respiration. In the adipose tissues from mice on a high-fat diet, expression of LSD1-target genes is reduced, compared with that in tissues from mice on a normal diet, which can be reverted by suppressing LSD1 function. Our data suggest a novel mechanism where LSD1 regulates cellular energy balance through coupling with cellular FAD biosynthesis. In response to environmental stimuli, epigenetic marks such as DNA and histone methylation may be dynamically added and removed for gene regulation during the transcriptional cycle [1] , [2] . Nutritional information may influence the epigenome by directly affecting the activities of epigenetic modifiers [3] . Notably, it has been reported that nutritional conditions in early life influence the susceptibility to chronic disorders, such as obesity and related metabolic diseases, later in life [4] , suggesting underlying epigenetic mechanisms [5] . Thus, elucidating how nutritional information is transferred to the epigenetic machinery for the regulation of cellular metabolism, and the formation of the long-term metabolic phenotype is of great interest. Lysine-specific demethylase-1 (LSD1, also known as KDM1A) is a member of the flavin-containing amine oxidase family that, in general, represses transcription by removing the methyl group from mono-methylated and di-methylated lysine 4 of histone H3 (H3K4) [6] . LSD1 is also involved in the demethylation of H3K9 when associated with some nuclear receptors [7] , and in the demethylation of non-histone proteins such as p53, Stat3 and Dnmt1 (ref. 8 , 9 , 10 ), suggesting its contribution to selective biological processes. Indeed, genetic ablation of LSD1 in mice causes embryonic lethality [11] , and LSD1-deficient embryonic stem cells had cell defects and global DNA hypomethylation [10] , consistent with the important functions of LSD1. Among numerous epigenetic factors, LSD1 is unique in that it utilizes flavin adenosine dinucleotide (FAD) as an essential cofactor for catalytic activities [12] . FAD serves as a coenzyme in many oxidative reactions including mitochondrial fatty acid β-oxidation and in the respiratory chain [13] . The majority of reported flavoenzymes localize to the mitochondria or cytoplasm, whereas LSD1 is one of a few flavoproteins in the nucleus. Another nuclear flavoprotein is apoptosis-inducing factor (AIF) that initially localizes to the mitochondrial inner membrane and translocates to the nucleus on oxidative stress or other proapoptotic stimuli, leading to DNA degradation [14] , suggesting that AIF may transfer the mitochondrial metabolic information to the nucleus [15] . However, the biological significance of FAD-dependent LSD1 activities in metabolic regulation remains unknown. In this study, we present direct evidence that the inhibition of LSD1, by short interfering RNA (siRNA)-mediated knockdown (KD) and by selective inhibitors, activates energy-expenditure genes by transcriptional and epigenetic mechanisms in adipocytes. Disruption of LSD1 function resulted in the de-repression of these genes leading to the activation of mitochondrial respiration and lipolysis in adipocytes. We further found that LSD1-mediated transcriptional repression is FAD-dependent, and that the disruption of cellular FAD synthesis exerted similar effects on the metabolic gene expression as the LSD1 inhibition. Importantly, the expression of LSD1-target genes was markedly repressed in high fat-exposed white adipose tissue (WAT), and could be reverted by LSD1 inhibition, indicating the involvement of LSD1 in metabolic adaptation in vivo . Our data shed light on an essential mechanism of energy utilization that might explain how cells determine their energy strategy depending on nutritional availability. LSD1 regulates energy-expenditure genes in adipocytes During our investigations, we found that both LSD1 and its essential partner BHC80 (ref. 16 ), showed relatively high expression levels in WAT among metabolic tissues in mice ( Fig. 1a ; Supplementary Fig. S1a ). In addition, adipogenic 3T3-L1 cells abundantly expressed BHC80, which was found to form a complex with LSD1 in these cells ( Fig. 1b ; Supplementary Fig. S1b,c ). During adipogenesis, an increase in mono-methylated H3K4 was observed, which is indicative of the active regulation of H3K4 methylation in these cells ( Supplementary Fig. S1d ). To address the role of LSD1 function in adipose cells, we performed microarray-based expression analyses in 3T3-L1 cells. We disrupted LSD1 function by using specific siRNAs for LSD1 and BHC80 ( Fig. 1c ), as well as by using an LSD1 inhibitor, tranylcypromine (TC, also known as trans-2-phenylcyclopropylamine) [17] , [18] , [19] , [20] , [21] , in adipocyte-differentiating 3T3-L1 cells. TC was initially identified as an inhibitor of monoamine oxidases (MAO) A and B [22] , and was demonstrated to be a potent inhibitor of LSD1 (refs 17 , 18 ). In agreement with the transcriptional repressive activities of LSD1, 198 probe sets were commonly induced 1.5-fold or more by LSD1-KD, BHC80-KD and TC treatment ( Fig. 1d ; Supplementary Data 1 ). Focusing on the probe sets upregulated by LSD1-KD, we found significant enrichment of the probe sets that were similarly upregulated by TC ( P =2.8×10 −56 by χ 2 test), while only a few were oppositely regulated ( Fig. 1e ). A similar tendency was observed for the co-target probes of LSD1-KD and BHC80-KD ( P =8.0×10 −8 by χ 2 test). To clarify the biological relevance of the co-target genes, we used Gene set enrichment analysis [23] ( Fig. 1f ). Considering the physiological function of adipocytes, we found that many of the co-target genes were related to lipid metabolism and mitochondrial oxidative phosphorylation (OXPHOS). On the other hand, 95 probe sets were commonly downregulated more than 1.5-fold by LSD1-KD, BHC80-KD and TC. However, GSEA analysis of the downregulated genes under LSD1 inhibition identified no significantly enriched gene sets associated with energy metabolism ( Fig. 1g ; Supplementary Data 2 ). 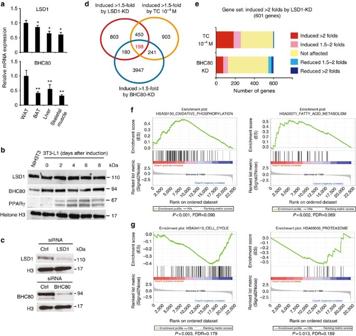Figure 1: Genome-wide analyses of LSD1-regulated genes in adipocytes. (a) Preferential expression of LSD1 and BHC80 in WAT. Expression ofLSD1andBHC80mRNAs in epididymal WAT, interscapular BAT, liver and skeletal muscle. 13-week old C57BL/6J mice were fasted for 16 h before tissue dissection. Quantitative RT–PCR values were normalized to the expression levels of the housekeeping36B4gene, and are shown as means±s.d. of four mice. *P<0.05, **P<0.01 versus WAT by Student'st-test. (b) The protein expression of LSD1 and BHC80 in adipogenic 3T3-L1 cells. The cells were subjected to adipogenic induction as described in Methods, and were collected at the indicated time points. (c) Specific siRNA-mediated knockdown of LSD1 and BHC80 in 3T3-L1 cells.In silicoanalysis, using mouse genome and EST databases, confirmed the target specificities of the siRNAs. For western blot analysis, protein samples were prepared 72 h after siRNA introduction. (d) Venn diagram of the genes induced 1.5-fold or more by LSD1-knockdown (KD), BHC80-KD or TC treatment. siRNA-introduced or TC-treated 3T3-L1 cells were subjected to adipogenic induction for 24 h. Control siRNA or vehicle-treated samples were used as controls. (e) Unidirectional effects of TC and BHC80-KD on LSD1-target genes. (f) Gene set enrichment analysis of commonly upregulated genes by LSD1-KD, BHC80-KD and TC treatment. In each panel, nominalP-values and false discovery rates (FDRs) are indicated. (g) Gene set enrichment analysis of commonly downregulated genes by LSD1-KD, BHC80-KD and TC treatment. Significantly enriched gene sets are shown. NominalP-values and FDRs are indicated. Figure 1: Genome-wide analyses of LSD1-regulated genes in adipocytes. ( a ) Preferential expression of LSD1 and BHC80 in WAT. Expression of LSD1 and BHC80 mRNAs in epididymal WAT, interscapular BAT, liver and skeletal muscle. 13-week old C57BL/6J mice were fasted for 16 h before tissue dissection. Quantitative RT–PCR values were normalized to the expression levels of the housekeeping 36B4 gene, and are shown as means±s.d. of four mice. * P <0.05, ** P <0.01 versus WAT by Student's t -test. ( b ) The protein expression of LSD1 and BHC80 in adipogenic 3T3-L1 cells. The cells were subjected to adipogenic induction as described in Methods, and were collected at the indicated time points. ( c ) Specific siRNA-mediated knockdown of LSD1 and BHC80 in 3T3-L1 cells. In silico analysis, using mouse genome and EST databases, confirmed the target specificities of the siRNAs. For western blot analysis, protein samples were prepared 72 h after siRNA introduction. ( d ) Venn diagram of the genes induced 1.5-fold or more by LSD1-knockdown (KD), BHC80-KD or TC treatment. siRNA-introduced or TC-treated 3T3-L1 cells were subjected to adipogenic induction for 24 h. Control siRNA or vehicle-treated samples were used as controls. ( e ) Unidirectional effects of TC and BHC80-KD on LSD1-target genes. ( f ) Gene set enrichment analysis of commonly upregulated genes by LSD1-KD, BHC80-KD and TC treatment. In each panel, nominal P -values and false discovery rates (FDRs) are indicated. ( g ) Gene set enrichment analysis of commonly downregulated genes by LSD1-KD, BHC80-KD and TC treatment. Significantly enriched gene sets are shown. Nominal P -values and FDRs are indicated. Full size image By quantitative RT–PCR analyses, we confirmed that important regulators of energy metabolism ( Fig. 2a ), such as PPARγ coactivator-1α (PGC-1α), pyruvate dehydrogenase kinase 4 (PDK4), protein kinase A regulatory subunit 2 alpha (RIIalpha) and adipose triglyceride lipase (ATGL), were significantly upregulated ( Fig. 2b,c; Supplementary Data 1 ). These gene products have been reported to have key roles in mitochondrial energy production and/or lipid mobilization [24] , [25] , [26] , [27] . Among them, elevated expression of PGC-1α is a hallmark of brown adipose tissue (BAT), which is specialized for consumptive metabolism for the purpose of thermogenesis [28] . Consistently, LSD1 inhibition induced the expression of fatty acid transporter 1 (FATP1), a critical regulator of BAT metabolism ( Fig. 2b,c ) [29] , [30] . The selective upregulation of the group of energy-expenditure genes was confirmed by the use of alternative siRNA against LSD1 ( Fig. 2d,e ). We also noticed that LSD1 inhibition did not affect the expression of the key adipogenic factors as well as the drivers of brown adipogenesis ( Supplementary Table S1 ). 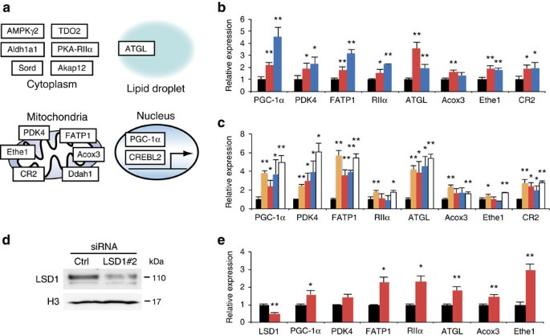Figure 2: LSD1 inhibition activates genes for energy expenditure and mitochondrial metabolism in adipocytes. (a) Summarized illustration of co-target genes. Co-target genes , associated with energy expenditure and mitochondrial metabolism, are shown with cellular localization of the gene products. (b) Expression levels of LSD1 target genes under LSD1-KD (red bars) and BHC80-KD (blue bars). Quantitative RT–PCR values were normalized to the expression levels of the36B4gene, and are shown as the fold difference against control siRNA-introduced samples (black bars). (c) Expression levels of LSD1 target genes after TC (orange bars) or SLIs (S2101 (red bars), S2107 (blue bars), S2111 (white bars)) treatment. TC and SLIs were used at the concentrations of 10−4M and 10−5M, respectively. Values are shown as the fold difference against vehicle-treated samples (black bars). (d) The knockdown of LSD1 using an alternative siRNA (LSD1#2). (e) The effect of LSD1 siRNA#2 on the expression of newly identified LSD1-target genes. Values are shown as the fold difference against control siRNA-introduced samples (black bars). All histogram data are means±s.d. of triplicate results. *P<0.05, **P<0.01 versus control by Student'st-test. Figure 2: LSD1 inhibition activates genes for energy expenditure and mitochondrial metabolism in adipocytes. ( a ) Summarized illustration of co-target genes. Co-target genes , associated with energy expenditure and mitochondrial metabolism, are shown with cellular localization of the gene products. ( b ) Expression levels of LSD1 target genes under LSD1-KD (red bars) and BHC80-KD (blue bars). Quantitative RT–PCR values were normalized to the expression levels of the 36B4 gene, and are shown as the fold difference against control siRNA-introduced samples (black bars). ( c ) Expression levels of LSD1 target genes after TC (orange bars) or SLIs (S2101 (red bars), S2107 (blue bars), S2111 (white bars)) treatment. TC and SLIs were used at the concentrations of 10 −4 M and 10 −5 M, respectively. Values are shown as the fold difference against vehicle-treated samples (black bars). ( d ) The knockdown of LSD1 using an alternative siRNA (LSD1#2). ( e ) The effect of LSD1 siRNA#2 on the expression of newly identified LSD1-target genes. Values are shown as the fold difference against control siRNA-introduced samples (black bars). All histogram data are means±s.d. of triplicate results. * P <0.05, ** P <0.01 versus control by Student's t -test. Full size image As TC is also a potent MAO inhibitor, we employed selective LSD1 inhibitors (SLIs) to discriminate whether the activation of the metabolic genes is attributable to specific inactivation of the enzymatic activity of LSD1. We used three SLIs, S2101, S2107 and S2111, which are structurally related to TC, but highly potent with substantially reduced affinity to MAOs ( Supplementary Fig. S2a ) [31] . All SLIs showed coherent effects against LSD1-target metabolic genes, suggesting a strong link between the enzymatic activity of LSD1 and energy metabolism ( Fig. 2c ). In addition, MAO inhibitors, pargyline and clorgyline [17] , did not activate LSD1-target genes at the tested concentrations ( Supplementary Fig. S2b ). Consistently, IC50 values of LSD1 and MAO inhibitors correlate well with the activation of LSD1-target genes by these drugs ( Supplementary Table S2 ). The expression microarray analysis, using the cells treated with SLIs, confirmed the selectivity of these drugs, and further emphasized the link between LSD1 enzymatic activity and metabolic gene regulation ( Supplementary Fig. S2c,d ). Collectively, these results indicate that LSD1 represses expression of the energy-expenditure genes in adipocytes. LSD1 epigenetically represses energy-expenditure genes To investigate the molecular mechanism of LSD1 action, we tested whether energy-expenditure genes are directly regulated by LSD1 in differentiating 3T3-L1 cells. Chromatin immunoprecipitation (ChIP) analysis revealed that LSD1 was specifically enriched near the transcription start site of the PGC-1 α promoter (sites 3 and 4) ( Fig. 3a ). Similarly, the selective occupancy of LSD1 was observed at the PDK4 , FATP1 and ATGL gene promoters but not at the actB gene promoter (encoding β-actin) ( Fig. 3b ). The enrichment of di/tri-methylated H3K4 as well as acetylated H3 was enhanced by LSD1-KD at LSD1-bound promoters, whereas the actB promoter remained unchanged ( Fig. 3c,d ). Moreover, Pdx1 gene, which is not expressed in adipose cells, showed enriched LSD1 occupancy and the increased H3K4 methylation after LSD1-KD, emphasizing the close relationship between LSD1 and H3K4 demethylation in energy-expenditure genes ( Fig. 3b,c ). Di-methylated H3K4 was enriched at the PGC-1 α promoter under the TC treatment ( Fig. 3e ), consistent with the inhibition of LSD1-dependent demethylation by TC. 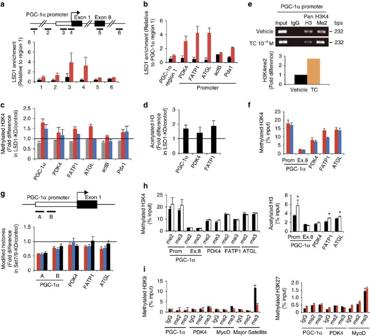Figure 3: Epigenetic repression of energy-expenditure genes by LSD1. After 24-hour adipogenic induction, 3T3-L1 cells were examined for LSD1 enrichment and histone modifications by ChIP–qPCR. Before the induction, cells were subjected to siRNA introduction or drug treatment, as specified below. Each ChIP–qPCR histogram indicates the mean±s.d. of triplicate results. (a) Localization of LSD1 at thePGC-1α gene locus. ChIP analyses were performed in 3T3-L1 cells after 24-hour adipogenic induction using anti-LSD1 antibody. Six indicated sites (1–6) were tested for qPCR amplification. Enrichment values were normalized to input, and shown as the fold difference relative to region 1. Control IgG (black bars), anti-LSD1 antibody (red bars). (b) LSD1 occupancy atPDK4,FATP1 ATGL,actBandPdx1gene promoters. LSD1 occupancy was calculated as the enrichment level relative toPGC-1α gene exon 8. Control IgG (black bars), anti-LSD1 antibody (red bars). (c) ChIP analyses of the target gene promoters using antibodies against mono- (grey bars), di- (red bars) and tri-methylated (blue bars) H3K4. The enrichment values are shown as the fold difference relative to control siRNA-introduced cells. (d) Histone H3 acetylation levels of LSD1-target promoters after LSD1-KD. (e) Enrichment of di-methylated H3K4 at thePGC-1α gene promoter in TC-treated cells. Three independent assays had similar results. (f) Di- (red bars) and tri-methylation (blue bars) levels of H3K4 on LSD1-regulated genes. Values indicate percentage of input DNA. (g) Histone modification levels of LSD1 target promoters after Set7/9-KD. The enrichment values of di- (red bars), tri- (blue bars) methylated H3K4 and acetylated H3 (black bars) are shown as the fold difference relative to control siRNA-introduced cells. (h) Effect of TSA treatment on H3K4 methylation (left panel) and H3 acetylation (right panel). Cells were cultured with vehicle (white bars) or with 100 nM TSA (black bars) before adipogenic induction. *P<0.05 versus vehicle by Student'st-test. (i) Repressive histone marks in LSD1-KD (red bars) and control (black bars) cells. ChIP experiments were done using antibodies against di- and tri-methylated H3K9 (left panel) and di- and tri-methylated H3K27 (right panel).MyoDgene and major satellite repeat were included as experimental controls. Figure 3: Epigenetic repression of energy-expenditure genes by LSD1. After 24-hour adipogenic induction, 3T3-L1 cells were examined for LSD1 enrichment and histone modifications by ChIP–qPCR. Before the induction, cells were subjected to siRNA introduction or drug treatment, as specified below. Each ChIP–qPCR histogram indicates the mean±s.d. of triplicate results. ( a ) Localization of LSD1 at the PGC-1 α gene locus. ChIP analyses were performed in 3T3-L1 cells after 24-hour adipogenic induction using anti-LSD1 antibody. Six indicated sites (1–6) were tested for qPCR amplification. Enrichment values were normalized to input, and shown as the fold difference relative to region 1. Control IgG (black bars), anti-LSD1 antibody (red bars). ( b ) LSD1 occupancy at PDK4 , FATP1 ATGL , actB and Pdx1 gene promoters. LSD1 occupancy was calculated as the enrichment level relative to PGC-1 α gene exon 8. Control IgG (black bars), anti-LSD1 antibody (red bars). ( c ) ChIP analyses of the target gene promoters using antibodies against mono- (grey bars), di- (red bars) and tri-methylated (blue bars) H3K4. The enrichment values are shown as the fold difference relative to control siRNA-introduced cells. ( d ) Histone H3 acetylation levels of LSD1-target promoters after LSD1-KD. ( e ) Enrichment of di-methylated H3K4 at the PGC-1 α gene promoter in TC-treated cells. Three independent assays had similar results. ( f ) Di- (red bars) and tri-methylation (blue bars) levels of H3K4 on LSD1-regulated genes. Values indicate percentage of input DNA. ( g ) Histone modification levels of LSD1 target promoters after Set7/9-KD. The enrichment values of di- (red bars), tri- (blue bars) methylated H3K4 and acetylated H3 (black bars) are shown as the fold difference relative to control siRNA-introduced cells. ( h ) Effect of TSA treatment on H3K4 methylation (left panel) and H3 acetylation (right panel). Cells were cultured with vehicle (white bars) or with 100 nM TSA (black bars) before adipogenic induction. * P <0.05 versus vehicle by Student's t -test. ( i ) Repressive histone marks in LSD1-KD (red bars) and control (black bars) cells. ChIP experiments were done using antibodies against di- and tri-methylated H3K9 (left panel) and di- and tri-methylated H3K27 (right panel). MyoD gene and major satellite repeat were included as experimental controls. Full size image We then investigated the mechanism of LSD1-mediated transcriptional repression. LSD1-regulated promoters were enriched with relatively high levels of methylated H3K4, consistent with their active transcription in adipose cells ( Fig. 3f ). The knockdown of H3K4 methyltransferase Set7/9 resulted in a partial reduction of methylated H3K4, suggesting that methylation equilibrium on these promoters was formed through active methylation/demethylation forces ( Fig. 3g ). Treatment of the cells with Trichostatin A (TSA), a HDAC inhibitor, induced histone H3 acetylation of the energy-expenditure genes without affecting H3K4 methylation status ( Fig. 3h ). This suggests that enhanced H3K4 methylation by LSD1 inhibition was not merely a reflection of active chromatin formation, but rather indicates the direct relationship between LSD1 function and H3K4 methylation on these promoters. Typical repressive histone marks, methylated H3K9 and H3K27, were detected only at background levels on LSD1-target promoters, and were not influenced by LSD1-KD ( Fig. 3i ). To assess promoter silencing by LSD1, reporter assays were performed in which the mouse PGC-1 α promoter was fused to the luciferase reporter gene (PGC-1α/Luc) ( Fig. 4a ). As expected, PGC-1α/Luc activity was induced by LSD1-KD and BHC80-KD ( Fig. 4b ). As well, TC and SLIs significantly activated the PGC-1 α promoter ( Fig. 4c,d ). We also examined the chromatin regulation of the PGC-1α/Luc transgene by LSD1. The ChIP assay confirmed that the transfected PGC-1α/Luc plasmid was engaged with histone H3, indicating the incorporation of the transgene into the nucleosome structure ( Fig. 4e ). TC treatment induced the increase of H3K4 di-methylation at the 5′ region of the transgenic PGC-1α promoter where LSD1 was bound ( Fig. 4f,g ). Thus, energy-expenditure genes are direct targets of the LSD1-mediated repression. 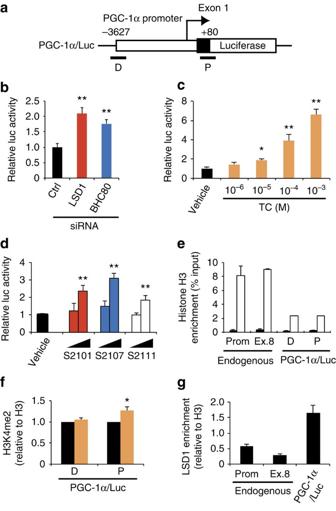Figure 4: Transcriptional repression ofPGC-1α promoter by LSD1. (a) Diagram of PGC-1α/Luc construct. Sites of ChIP–qPCR primers are indicated as D (distal) and P (proximal). (b) Effects of LSD1-KD and BHC80-KD onPGC-1α promoter activity. After the introduction of indicated siRNAs, 3T3-L1 cells were transfected with a PGC-1α/Luc plasmid and an internal control pRL-TK construct. Luciferase activities were measured at 24 h after the adipogenic induction. (c,d) Effects of LSD1 inhibitors onPGC-1α gene promoter activity. TC (c) was used at the indicated concentrations whereas SLIs (d) were used at 10−6and 10−5M. Reporter-introduced cells were treated with indicated drugs for 24 h before the adipogenic induction. (e) Chromatin formation on transfected reporter plasmid. Pan-histone H3 (white bars) and control IgG (black bars) levels were analysed both on endogenous and transgenicPGC-1α promoter. (f) H3K4 di-methylation level of the reporter vector after vehicle (black bars) or 10−4M TC (orange bars) treatment. Values are normalized to the enrichment level of panH3. (g) LSD1-binding on the reporter vector. Values are normalized to the enrichment level of panH3. Values are mean±s.d. of triplicate samples. *P<0.05, **P<0.01 versus control siRNA or vehicle by Student'st-test. Figure 4: Transcriptional repression of PGC-1 α promoter by LSD1. ( a ) Diagram of PGC-1α/Luc construct. Sites of ChIP–qPCR primers are indicated as D (distal) and P (proximal). ( b ) Effects of LSD1-KD and BHC80-KD on PGC-1 α promoter activity. After the introduction of indicated siRNAs, 3T3-L1 cells were transfected with a PGC-1α/Luc plasmid and an internal control pRL-TK construct. Luciferase activities were measured at 24 h after the adipogenic induction. ( c , d ) Effects of LSD1 inhibitors on PGC-1 α gene promoter activity. TC ( c ) was used at the indicated concentrations whereas SLIs ( d ) were used at 10 −6 and 10 −5 M. Reporter-introduced cells were treated with indicated drugs for 24 h before the adipogenic induction. ( e ) Chromatin formation on transfected reporter plasmid. Pan-histone H3 (white bars) and control IgG (black bars) levels were analysed both on endogenous and transgenic PGC-1 α promoter. ( f ) H3K4 di-methylation level of the reporter vector after vehicle (black bars) or 10 −4 M TC (orange bars) treatment. Values are normalized to the enrichment level of panH3. ( g ) LSD1-binding on the reporter vector. Values are normalized to the enrichment level of panH3. Values are mean±s.d. of triplicate samples. * P <0.05, ** P <0.01 versus control siRNA or vehicle by Student's t -test. Full size image LSD1 inhibition activates mitochondrial metabolism As the LSD1 inhibition resulted in the expression of energy-expenditure genes associated with mitochondrial metabolism, we sought to determine the metabolic consequences of LSD1-inhibited conditions. To address this, LSD1-inhibited differentiating 3T3-L1 cells were stained with JC-1, a fluorescent dye that binds to the mitochondrial inner membrane showing green fluorescence (FL1; mitochondrial mass) and forms red-fluorescent aggregates depending on the membrane potential (FL2; respiratory activity) [32] . Flow cytometric analyses of JC-1-stained cells revealed that LSD1-KD significantly augmented the mitochondrial membrane potential with an elevated FL2/FL1 ratio that represents the respiratory activity relative to the mitochondrial surface area ( Fig. 5a ). TC and SLIs also potently augmented the mitochondrial metabolism although pargyline did not ( Fig. 5b ; Supplementary Fig. 3a,b ). The activated oxidative metabolism by LSD1 inhibition was also confirmed by measuring the OXPHOS capacity using a XF24 Extracellular Flux Analyzer (Seahorse). The maximum OXPHOS capacity was dramatically potentiated by LSD1-KD ( Fig. 5c ). On the other hand, glycolytic activity, as determined by cellular lactate production, was not significantly affected by either LSD1-KD or TC ( Supplementary Fig. S3c,d ). 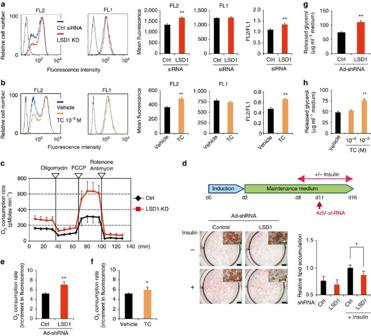Figure 5: LSD1 inhibition enhances mitochondrial metabolism in adipocytes. Mitochondrial energy metabolism was assessed in differentiating 3T3-L1 cells under LSD1-KD (a) and TC treatment (b). siRNA-introduced or drug-treated cells were subjected to adipogenic induction for 24 h, and were stained with JC-1 followed by flow cytometric analyses. Red fluorescent JC-1 aggregates (FL2) and green fluorescent monomers (FL1) were measured. Hatched histograms indicate the unstained control samples. Each histogram shows the representative result of triplicate samples. (c) The effect of LSD1-KD on the OXPHOS capacity of differentiating 3T3-L1 cells. OXPHOS activity was determined by measuring the OCR using the XF24 Analyzer. During the real-time measurement, respiratory chain inhibitors were added to the culture at the indicated time points. Values are means±s.d. of five assay wells at each time point. (d) LSD1-KD reduces lipid accumulation in insulin-stimulated adipocytes. Differentiated 3T3-L1 cells were cultured in the absence or presence of insulin, followed by adenovirus-mediated introduction of LSD1 shRNA (Ad-shLSD1) or control (Ad-sh-ctrl). Cellular lipid was analysed at 4 days after infection. Values are means±s.d. of five mice. Scale bars in the whole-well and magnified images indicate 5 mm and 50 μm, respectively. (e,f) The effects of LSD1-KD and TC treatment on the OCR in mature 3T3-L1 adipocytes. Insulin-stimulated adipocytes were treated with shRNA-containing adenoviruses (control or LSD1,e) or 10−4M TC (f), and cultured for 4 days. OCR was determined using the Oxygen Biosensor System, and was calculated as the fold increase during 30 min-measurement. (g,h) Enhanced lipolysis in LSD1-inhibited adipocytes. Insulin-stimulated mature 3T3-L1 adipocytes were infected with shRNA-containing adenovirus (g) or were treated with TC (h), and cultured for 4 days. All values (except for those inc) are means±s.d. of three independent samples. *P<0.05, **P<0.01 versus control siRNA, control shRNA or vehicle by Student'st-test Figure 5: LSD1 inhibition enhances mitochondrial metabolism in adipocytes. Mitochondrial energy metabolism was assessed in differentiating 3T3-L1 cells under LSD1-KD ( a ) and TC treatment ( b ). siRNA-introduced or drug-treated cells were subjected to adipogenic induction for 24 h, and were stained with JC-1 followed by flow cytometric analyses. Red fluorescent JC-1 aggregates (FL2) and green fluorescent monomers (FL1) were measured. Hatched histograms indicate the unstained control samples. Each histogram shows the representative result of triplicate samples. ( c ) The effect of LSD1-KD on the OXPHOS capacity of differentiating 3T3-L1 cells. OXPHOS activity was determined by measuring the OCR using the XF24 Analyzer. During the real-time measurement, respiratory chain inhibitors were added to the culture at the indicated time points. Values are means±s.d. of five assay wells at each time point. ( d ) LSD1-KD reduces lipid accumulation in insulin-stimulated adipocytes. Differentiated 3T3-L1 cells were cultured in the absence or presence of insulin, followed by adenovirus-mediated introduction of LSD1 shRNA (Ad-shLSD1) or control (Ad-sh-ctrl). Cellular lipid was analysed at 4 days after infection. Values are means±s.d. of five mice. Scale bars in the whole-well and magnified images indicate 5 mm and 50 μm, respectively. ( e , f ) The effects of LSD1-KD and TC treatment on the OCR in mature 3T3-L1 adipocytes. Insulin-stimulated adipocytes were treated with shRNA-containing adenoviruses (control or LSD1, e ) or 10 −4 M TC ( f ), and cultured for 4 days. OCR was determined using the Oxygen Biosensor System, and was calculated as the fold increase during 30 min-measurement. ( g , h ) Enhanced lipolysis in LSD1-inhibited adipocytes. Insulin-stimulated mature 3T3-L1 adipocytes were infected with shRNA-containing adenovirus ( g ) or were treated with TC ( h ), and cultured for 4 days. All values (except for those in c ) are means±s.d. of three independent samples. * P <0.05, ** P <0.01 versus control siRNA, control shRNA or vehicle by Student's t -test Full size image To characterize the metabolic properties of mature adipocytes under LSD1 inhibition, we used an adenovirus-based method to introduce short hairpin RNA (shRNA) into mature 3T3-L1 adipocytes ( Supplementary Fig. S4a ). LSD1-KD resulted in the significant reduction of lipid accumulation only when the lipogenesis was enhanced under insulin-stimulated condition ( Fig. 5d ). Consistently, insulin-induced repression of energy-expenditure genes was attenuated by LSD1-KD ( Supplementary Fig. 4b ). In the insulin-stimulated adipocytes, oxidative metabolism was activated by LSD1-KD and TC treatment ( Fig. 5e,f ). LSD1 inhibition also reduced lipid accumulation in differentiating adipocytes ( Supplementary Fig. 4c,d ). Thus, LSD1 suppresses mitochondrial energy metabolism in mature adipocytes depending on the cellular energy condition. Because we observed the activated mitochondrial metabolism and the reduced lipid accumulation in LSD1-inhibited states in adipocytes, we checked whether lipolysis was also activated ( Fig. 5g,h ). Both LSD1-KD and TC treatment in insulin-stimulated mature 3T3-L1 adipocytes significantly augmented the lipolytic activity. Several types of triglyceride lipases are involved in lipolysis and are mainly controlled by the PKA-mediated signal cascade [24] , [25] . Consistently, ATGL and a number of PKA-associated genes were upregulated in LSD1-inhibited cells ( Fig. 2a–c ; Supplementary Data 1 ). Collectively, these results suggest that LSD1 suppresses energy expenditure by inhibiting mitochondrial respiration and lipid mobilization in adipocytes. Loss of FAD attenuates the gene regulatory activity of LSD1 To investigate the biological importance of FAD-dependent LSD1 activities, we examined whether cellular FAD synthesis affects the expression of the LSD1-target genes involved in energy metabolism. The biosynthetic pathway from riboflavin to FAD is composed of two enzymes, riboflavin kinase (RFK) and FAD synthetase (FADS) [33] ( Fig. 6a ). The siRNA-mediated knockdown of these two genes resulted in a mild reduction of the cellular FAD content in 3T3-L1 cells whereas RFK-KD showing the stronger effect, as assessed by two different methods ( Supplementary Fig. S5a,b ). Expression of most LSD1-target genes was increased by RFK-KD while FADS-KD did not affect PGC-1 α expression, in agreement with their effects on FAD production ( Fig. 6b ; Supplementary Fig. S5c ). These results imply that RFK is the rate-limiting enzyme in the FAD biosynthetic process. It might be analogous to the case of the NAD + (nicotinamide adenine dinucleotide) synthetic pathway in which Nampt, the first enzyme of the process, strongly affects the cellular NAD + pool [34] . To elucidate the substantial overlap in the target genes, expression microarray analysis was performed using LSD1-KD and RFK-KD cells ( Fig. 6c ). A total of 132 genes were commonly induced more than twofold compared with the control under both knockdown conditions. In addition, as we focused on the probe sets upregulated by LSD1-KD, we found significant enrichment of the probe sets that were similarly upregulated by RFK-KD ( P =3.5×10 −47 by χ 2 test), compared with those oppositely regulated ( Fig. 6d ). 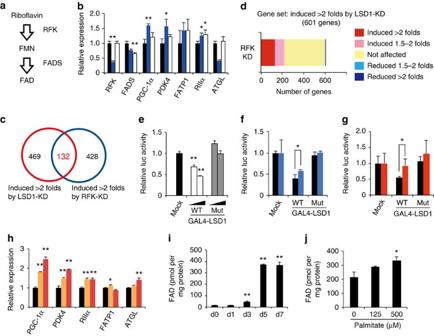Figure 6: Inhibition of cellular FAD synthesis blocks LSD1-mediated repression of energy-expenditure genes. (a) Biosynthesis pathway of FAD in mammalian cells. Flavin mononucleotide (FMN). (b) Effect of the disruption of FAD synthesis on LSD1-target genes. RFK- (blue bars) or FADS- (white bars) knockdown 3T3-L1 cells were induced to differentiate for 24 h, followed by RNA extraction and quantitative RT–PCR. Values are shown as the fold difference against control siRNA-introduced samples (black bars). *P<0.05, **P<0.01 versus control siRNAs by Student'st-test. (c) Venn diagram of the probe sets induced by LSD1-KD and RFK-KD. (d) Unidirectional effects of RFK-KD on LSD1-target genes. (e) Effect of wild-type or FAD-binding mutant-type LSD1 on promoter activity. GAL4-fused LSD1-expressing plasmid (0.1 or 0.5 μg) was transfected into 293T cells, together with the GAL4x5-containing luciferase reporter construct. **P<0.01 versus GAL4 mock by Student'st-test. (f) Effect of RFK-KD on LSD1-mediated transcriptional repression. Control (black bars) or RFK (blue bars) siRNA-introduced 3T3-L1 cells were transfected with indicated GAL4 plasmids 48 h before the luciferase measurement. *P<0.05 between indicated conditions by Student'st-test. (g) Effect of lumiflavin treatment on LSD1-mediated transcriptional repression. 3T3-L1 cells were exposed to vehicle (black bars) or 50 μM lumiflavin (red bars) 48 h before the luciferase measurement. (h) Effect of lumiflavin on endogenous LSD1-target genes. Differentiating 3T3-L1 cells were exposed to vehicle (black bars), 25 μM (orange bars) or 50 μM (red bars) lumiflavin for 24 h and were subjected to RNA analyses. (i) Increase of FAD concentration during adipogenic differentiation of 3T3-L1 cells. **P<0.01 versus day 0 by Student'st-test. (j) Increase of FAD concentration after 24-hour palmitate exposure in mature 3T3-L1 adipocytes (day 7). Values are normalized to the protein concentration. *P<0.05 versus control by Student'st-test. All histogram values are means±s.d. of three independent samples. Figure 6: Inhibition of cellular FAD synthesis blocks LSD1-mediated repression of energy-expenditure genes. ( a ) Biosynthesis pathway of FAD in mammalian cells. Flavin mononucleotide (FMN). ( b ) Effect of the disruption of FAD synthesis on LSD1-target genes. RFK- (blue bars) or FADS- (white bars) knockdown 3T3-L1 cells were induced to differentiate for 24 h, followed by RNA extraction and quantitative RT–PCR. Values are shown as the fold difference against control siRNA-introduced samples (black bars). * P <0.05, ** P <0.01 versus control siRNAs by Student's t -test. ( c ) Venn diagram of the probe sets induced by LSD1-KD and RFK-KD. ( d ) Unidirectional effects of RFK-KD on LSD1-target genes. ( e ) Effect of wild-type or FAD-binding mutant-type LSD1 on promoter activity. GAL4-fused LSD1-expressing plasmid (0.1 or 0.5 μg) was transfected into 293T cells, together with the GAL4x5-containing luciferase reporter construct. ** P <0.01 versus GAL4 mock by Student's t -test. ( f ) Effect of RFK-KD on LSD1-mediated transcriptional repression. Control (black bars) or RFK (blue bars) siRNA-introduced 3T3-L1 cells were transfected with indicated GAL4 plasmids 48 h before the luciferase measurement. * P <0.05 between indicated conditions by Student's t -test. ( g ) Effect of lumiflavin treatment on LSD1-mediated transcriptional repression. 3T3-L1 cells were exposed to vehicle (black bars) or 50 μM lumiflavin (red bars) 48 h before the luciferase measurement. ( h ) Effect of lumiflavin on endogenous LSD1-target genes. Differentiating 3T3-L1 cells were exposed to vehicle (black bars), 25 μM (orange bars) or 50 μM (red bars) lumiflavin for 24 h and were subjected to RNA analyses. ( i ) Increase of FAD concentration during adipogenic differentiation of 3T3-L1 cells. ** P <0.01 versus day 0 by Student's t -test. ( j ) Increase of FAD concentration after 24-hour palmitate exposure in mature 3T3-L1 adipocytes (day 7). Values are normalized to the protein concentration. * P <0.05 versus control by Student's t -test. All histogram values are means±s.d. of three independent samples. Full size image Earlier studies have identified the 'GxGxxG' sequence as a FAD-binding consensus, one that is frequently present in FAD-dependent oxidases [35] ( Supplementary Fig. S5d ). To test whether FAD-binding is required for LSD1-mediated transcriptional repression, we point-mutated The 'GxGxxG' motif located at the amino-terminal side to the catalytic domain of LSD1. Structural modelling of LSD1 predicted that these mutations would deteriorate the LSD1/FAD interaction without affecting the overall folding of the protein [36] ( Supplementary Fig. S5e,f ). In the GAL4 reporter assay, wild-type LSD1 (GAL4-LSD1wt) suppressed the luciferase activities in a dose-dependent manner, whereas FAD binding-defective LSD1 (GAL4-LSD1mut) did not ( Fig. 6e ). We then tested whether cellular FAD production directly affects the repressive activity of LSD1. When FAD production was impaired by RFK-KD in 3T3-L1 cells, transcriptional repression by GAL4-LSD1wt was partly abolished ( Fig. 6f ). We also used lumiflavin, a riboflavin analogue that antagonizes the riboflavin transport into the cells [37] , which reduced the cellular FAD content ( Supplementary Fig. S5g ). LSD1 function was abrogated when lumiflavin was added to the culture medium ( Fig. 6g ). More importantly, the expression of endogenous LSD1 target genes was elevated after lumiflavin treatment ( Fig. 6h ). Lumiflavin also caused the reduction of LSD1 protein without affecting the messenger RNA level ( Supplementary Fig. S5h ), raising the possibility that LSD1 protein might be unstable when it is not bound to FAD. Taken together, these results suggest that LSD1 transcriptionally controls energy metabolism in a cellular FAD-dependent manner. To address whether the metabolic environment affects LSD1 activities, we examined the cellular FAD levels under the lipogenic conditions in 3T3-L1 cells. Interestingly, cellular FAD content remarkably increased during the adipogenic differentiation ( Fig. 6i ). In addition, palmitate exposure, which has been shown to facilitate lipid storage and suppress PGC-1α expression [38] , [39] , also led to an increase of FAD content in mature 3T3-L1 adipocytes ( Fig. 6j ). During the adipogenesis, the expression of LSD1-target genes including PGC-1α, PDK4 and FATP1 were increased, possibly reflecting their importance in adipocyte function ( Supplementary Fig. S6a ). The elevated FAD level may account for the activation of FAD-demanding processes such as fatty acid oxidation and TCA cycle on adipogenic differentiation. Palmitate exposure slightly reduced the expression levels of these genes, although not statistically significant ( Supplementary Fig. S6b ). The FAD content in the epididymal WAT from normal-diet (ND)- and high-fat-diet (HFD)-fed mice was measured, but no significant difference was found ( Supplementary Fig. S6c ). In this experiment, FAD concentration was about ten times lower than that of cultured adipocytes, possibly reflecting the difference in the magnitude of oxidative stress or the instability of FAD in tissue samples. The results show that the FAD content fluctuates depending on the cellular metabolic status, but further study is necessary to elucidate how FAD is utilized in different biological processes in the cell. Effect of LSD1 inhibition on gene expression in obese WAT To address the LSD1-dependent metabolic gene regulation in vivo , we performed gene-expression analyses in normal and obese adipose tissues of mice. Seven-week old C57BL/6J mice were fed a HFD for six weeks and acquired an obese state. Interestingly, in the adipose tissues of HFD-fed mice, the expression of LSD1 and BHC80 was markedly elevated compared with ND controls ( Fig. 7a,b ). In addition, the expression of the LSD1 target genes such as PGC-1 α, PDK4 and FATP1 was significantly reduced in the obese WAT tissues ( Fig. 7c ), indicating an inverse correlation with LSD1/BHC80 expression. 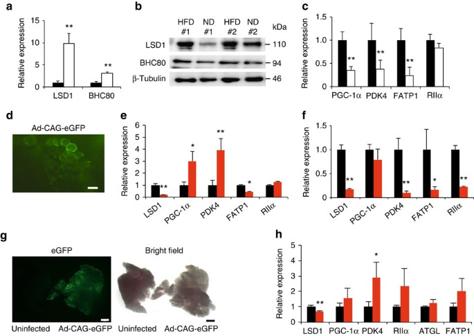Figure 7: Inhibition of LSD1 induces energy-expenditure genes in obese adipose tissues. (a,b) Expression of LSD1 and BHC80 in epididymal WAT from ND (black bars) and HFD- (white bars) fed mice. After a 16-hour fasting period, epididymal WAT was collected, and the total RNA was used for quantitative RT–PCR (a). The expression level of the36B4gene was used as the internal control. Protein levels are shown by western blot analysis (b). (c) Expression of LSD1 target genes in ND- (black bars) and HFD- (white bars) fed mice. Values are means±s.d. of four mice, and are shown as fold changes relative to ND-fed mice. **P<0.01 versus ND-fed mice by Student'st-test. (d) Efficient introduction of adenovirus vector into cultured WAT. Adenovirus vector, Ad-CAG-eGFP was introduced into isolated epididymal WAT, and the eGFP expression was analysed by fluorescence microscopy. Scale bar indicates 50 μm. (e,f) Expression of energy-expenditure genes after adenovirus-mediated knockdown ofLSD1gene in cultured WATex vivo. Epididymal WAT was dissected from either HFD- (e) or ND-fed mice (f), followed by the infection of adenoviruses, Ad-shLSD1 (red bars) or Ad-sh control (black bars). (g) Efficient introduction of adenoviral vectors into epididymal WATin vivo. Adenovirus vectors carrying theeGFPgene (Ad-CAG-eGFP) was injected into epididymal WAT after incising the outer coat of mice. Four days later, tissues were isolated for the microscopic analysis. Scale bar indicates 2 mm. (h) Expression of energy-expenditure genes after adenovirus-mediated reduction of LSD1 in epididymal WATin vivo. Control (black bars) or LSD1 (red bars) shRNA-carrying adenoviruses were directly injected into epididymal WAT of HFD-fed mice 4 days before tissue isolation. Values are means±s.d. of triplicate samples. *P<0.05, **P<0.01 versus control shRNA by Student'st-test. Figure 7: Inhibition of LSD1 induces energy-expenditure genes in obese adipose tissues. ( a , b ) Expression of LSD1 and BHC80 in epididymal WAT from ND (black bars) and HFD- (white bars) fed mice. After a 16-hour fasting period, epididymal WAT was collected, and the total RNA was used for quantitative RT–PCR ( a ). The expression level of the 36B4 gene was used as the internal control. Protein levels are shown by western blot analysis ( b ). ( c ) Expression of LSD1 target genes in ND- (black bars) and HFD- (white bars) fed mice. Values are means±s.d. of four mice, and are shown as fold changes relative to ND-fed mice. ** P <0.01 versus ND-fed mice by Student's t -test. ( d ) Efficient introduction of adenovirus vector into cultured WAT. Adenovirus vector, Ad-CAG-eGFP was introduced into isolated epididymal WAT, and the eGFP expression was analysed by fluorescence microscopy. Scale bar indicates 50 μm. ( e , f ) Expression of energy-expenditure genes after adenovirus-mediated knockdown of LSD1 gene in cultured WAT ex vivo . Epididymal WAT was dissected from either HFD- ( e ) or ND-fed mice ( f ), followed by the infection of adenoviruses, Ad-shLSD1 (red bars) or Ad-sh control (black bars). ( g ) Efficient introduction of adenoviral vectors into epididymal WAT in vivo . Adenovirus vectors carrying the eGFP gene (Ad-CAG-eGFP) was injected into epididymal WAT after incising the outer coat of mice. Four days later, tissues were isolated for the microscopic analysis. Scale bar indicates 2 mm. ( h ) Expression of energy-expenditure genes after adenovirus-mediated reduction of LSD1 in epididymal WAT in vivo . Control (black bars) or LSD1 (red bars) shRNA-carrying adenoviruses were directly injected into epididymal WAT of HFD-fed mice 4 days before tissue isolation. Values are means±s.d. of triplicate samples. * P <0.05, ** P <0.01 versus control shRNA by Student's t -test. Full size image To verify the direct relationship between LSD1 function and its target gene expression in obese adipose tissues, we employed the ex vivo culture of epididymal WAT in combination with adenovirus-mediated depletion of LSD1. We dissected adipose tissues from HFD-fed obese mice, and analysed the metabolic gene expression, 3 days after adenovirus introduction (at a multiplicity of infection (MOI) of 1.5×10 8 pfu dissected tissues −1 ) ( Fig. 7d ). In agreement with the above data, the loss of LSD1 increased the expression of some energy-expenditure genes such as PGC-1 α and PDK4 in obese adipose tissues ( Fig. 7e ). Interestingly, when tissues from ND-fed mice were used, LSD1-KD did not induce energy-expenditure gene expression suggesting the energetic state-dependent action of LSD1 ( Fig. 7f ). To further characterize the role of LSD1 in obese adipose tissues in vivo , we directly introduced the LSD1 shRNAs-expressing adenovirus into epididymal WAT (at a MOI of 5×10 8 pfu per mouse). Our repeated experiments using adenoviruses carrying the EGFP gene or LSD1 shRNAs showed the efficient introduction of exogenous gene into visceral adipose tissues ( Fig. 7g ). In agreement with the ex vivo studies, LSD1-KD in vivo induced relatively small but constant activation of the energy-expenditure genes in obese WAT without any evident tissue/cell defects ( Fig. 7h ). Thus, LSD1 represses energy-expenditure genes in adipose tissues, possibly participating in the establishment of the metabolic phenotypes in vivo . To evaluate the effect of TC administration on diet-induced obesity and the expression of energy-expenditure genes in adipose tissues in vivo , C57BL/6J mice were fed a HFD for six weeks in combination with an alternate-day administration of TC (10 mg per kg body weight) (HFD/TC) or PBS (HFD/PBS). HFD/TC mice showed markedly lower body weight and fat mass compared with the HFD/PBS-mice, with an improvement of the systemic lipid handling ( Supplementary Fig. S7a-d ). There was no difference in food intake among the groups ( Supplementary Fig. S7e ), and there were no abnormal behaviour or neurological symptoms in the TC-treated mice. Importantly, TC treatment induced the expression of PGC-1 α and other LSD1 targets as well as BAT marker UCP-1 in the epididymal WAT of the HFD/TC mice ( Supplementary Fig. S7f ). Collectively, these data further reinforce our finding that LSD1 is involved in the metabolic gene regulation. One of the key factors in formulating an energy strategy is environmental information such as nutritional availability. As many metabolism-associated genes are epigenetically regulated [40] , nutrient-driven epigenetic factors may have important roles in forming metabolic phenotypes [3] . LSD1 is a unique demethylase that does not contain the jumonji domain but as a flavoenzyme does have the FAD-dependent amine oxidase domain [1] . Our present study clearly indicates that LSD1 negatively regulates energy expenditure that can be reversed by inhibiting LSD1 function and FAD biosynthesis ( Fig. 8 ). Cellular FAD potentiates LSD1 to repress energy-expenditure genes such as PGC-1 α through H3K4 demethylation in adipocytes where excess energy is stored as triglycerides. Moreover, our experiments using mature adipocytes and isolated adipose tissues revealed the metabolic state-dependent effects of LSD1 inhibition. Thus, the transcriptional and epigenetic regulation by FAD-dependent LSD1 may be central in nutrient-driven metabolic adaptation. 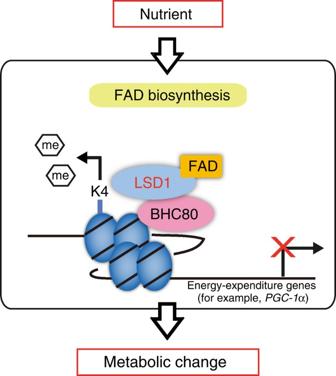Figure 8: Schematic model of LSD1 function in the metabolic gene regulation. Schematic model for the epigenetic regulation of energy metabolism by LSD1. FAD-dependent LSD1 facilitates metabolic changes through the repression of energy-expenditure genes via H3K4 demethylation. This pathway may be influenced by nutrients and/or fluctuating FAD level, implicating the link between energetic information and the epigenome. Figure 8: Schematic model of LSD1 function in the metabolic gene regulation. Schematic model for the epigenetic regulation of energy metabolism by LSD1. FAD-dependent LSD1 facilitates metabolic changes through the repression of energy-expenditure genes via H3K4 demethylation. This pathway may be influenced by nutrients and/or fluctuating FAD level, implicating the link between energetic information and the epigenome. Full size image In this study, we identified a set of energy expenditure-associated genes as direct targets of LSD1-mediated repression. We focused on the genes that were commonly induced by LSD1-KD, BHC80-KD and TC treatment. This criterion increased the likelihood of picking up genes that were directly regulated through H3K4 demethylation by LSD1, because BHC80 is reportedly the LSD1 partner required for H3K4 demethylation-dependent repression, and TC irreversibly inhibits the catalytic activity of LSD1 (refs 16 , 17 ). This finding was further confirmed by the use of SLIs with minimized nonspecific effects. Our microarray results also revealed the non-overlapping effects of LSD1-KD and BHC80-KD on the genome-wide expression profile. This suggests that in many cases, LSD1 and BHC80 regulate gene expression independently, and that BHC80 is dispensable for LSD1 function other than H3K4 demethylation. In fact, it is reported that BHC80 recognizes H3K4 to facilitate the demethylation by LSD1 (ref. 16 ), and only a fraction of LSD1 was associated with BHC80 in our experiment ( Supplementary Fig. S1c ). It is also noteworthy that reported phenotypes of LSD1 - and BHC80 -KO mice are distinctively different, indicating the non-overlapping biological function of these genes [11] , [41] . Mechanistically, LSD1 disruption induced moderate enrichment of methylated H3K4 on actively transcribed promoters. Histone methylation status can be determined by the equilibrium of methylating and demethylating forces, and, in many cases, LSD1 demethylation activity is counteracted by the lysine methyltransferase Set7/9 (refs 9 , 10 ). Interestingly, a previous report has shown that glucose-dependent induction of NF-κB gene expression was coincident with Set7/9-dependent H3K4 methylation, and was counteracted by LSD1, implying the possible involvement of Set7/9 in the metabolic gene regulation [42] . In our study, Set7/9-KD resulted in the partial reduction of H3K4 demethylation at LSD1-target promoters ( Fig. 3g ). Thus, it is possible that LSD1 fine-tunes the expression of metabolic genes so that the cellular energy balance can be properly maintained. We found in this study that the restriction of cellular FAD availability weakened the LSD1-dependent transcriptional repression of energy-expenditure genes. LSD1, like other flavoenzymes, requires FAD for its catalytic activity and converts it into the reduced form, FADH 2 (ref. 43 ). The catalytic activity of LSD1 may be directly connected to the cellular metabolic state via the fluctuation of the FAD/FADH 2 ratio depending on the FAD oxidation processes such as fatty acid β-oxidation and the TCA cycle. Another intriguing possibility is that a physical association between the LSD1 and FAD production machinery determines the LSD1 activities. Indeed, a recent study identified the existence of RFK in the protein complex containing TNFα receptor-1, in which RFK seemed to directly provide NADPH oxidase with FAD, facilitating the TNFα signalling [44] . Such a mechanism might explain why even a small reduction in FAD content in RFK-KD and lumiflavin-treated cells was sufficient for the LSD1 inhibition. In mitochondria, where the majority of FAD production occurs, flavoenzymes may stably associate with FAD even under FAD-reduced conditions [33] . As the FAD reserve for nuclear flavoenzymes is relatively small, their enzymatic activity could be highly sensitive to FAD restriction. It is of great interest that FAD-dependent LSD1-mediated demethylation may be analogous to, but clearly distinct from, NAD + -dependent Sirtuin 1 (Sirt1)-mediated deacetylation. Sirt1 is the orthologue of yeast Sir2 histone deacetylase, and promotes mitochondrial activation that contributes to calorie restriction-induced metabolic adaptation [45] . Regarding the regulation of the PGC-1α function, Sirt1 activates PGC-1α protein by deacetylating its lysine residue [46] , whereas LSD1 negatively regulates the expression of the PGC-1 α gene. Such opposing functions of LSD1 and Sirt1 suggest the existence of reciprocal switches for energy homeostasis in which FAD and NAD + serve as coenzymatic sensors. Aberration of cellular energy metabolism is associated with a wide range of multifactor and/or polygenic diseases including obesity-associated diseases, neurological disorders and cancer [47] , [48] , [49] . As epigenetic mechanisms are often linked to the pathogenesis of these diseases, the epigenetic factors responsible would be attractive as pharmacological therapeutic targets [5] , [50] , [51] . Our study depicts a novel mechanism of the crosstalk between energy metabolism and epigenetic gene regulation in which the FAD-dependent LSD1 activity regulates energy-expenditure genes. Thus, LSD1 inhibitors may be a new class of epigenetic drugs that can therapeutically benefit a wide range of metabolic disorders. Reagents and antibodies Tranylcypromine hydrochloride, pargyline hydrochloride and lumiflavin were purchased from Sigma. Clorgyline hydrochloride was purchased from MP Biomedicals. The compounds S2101, S2107 and S2111 were synthesized, as previously described [31] . JC-1 was purchased from Molecular Probes. The antibodies used were anti-LSD1 (Abcam, 1:500), anti-mono-methylated histone H3K4 (Abcam, 1:500), anti-di-methylated histone H3K4 (Millipore, 1:500), anti-tri-methylated histone H3K4 (Millipore, 1:500), anti-acetylated histone H3 (Millipore), anti-pan histone H3 (Abcam, 1:2000), anti-di-methylated histone H3K9 (Millipore), anti-tri-methylated histone H3K9 (Millipore), anti-di-methylated histone H3K27 (Millipore), and anti-tri-methylated histone H3K27 (Millipore). Anti-BHC80 antibodies (1:500) were a generous gift from Dr Tadashi Baba (Tsukuba University, Japan) [52] . Antibodies without dilution factors were only used for ChIP experiments. The amount of antibodies used is described here. Cell culture Mouse 3T3-L1, C3H10T1/2 cells, and human 293T cells were cultured in DMEM (Sigma) supplemented with 10% (v/v) heat-inactivated fetal bovine serum and penicillin/streptomycin. Adipogenic induction of 3T3-L1 cells was done by a standard method [53] . Post-confluent cells were exposed to adipogenic induction reagents including 0.5 mM 3-isobutyl-1-methylxanthine (Merck), 1 μM dexamethasone (Wako) and 5 μg ml −1 insulin (bovine pancreas, Sigma). For the experiments using differentiating adipocytes, cells were collected at 24 h after induction whereas for mature adipocytes, induction medium was replaced with maintenance medium after a 48-h-induction. Lipid accumulation was assessed by oil red O staining. For lipid quantification, oil red O was extracted with 2-propanol and was subjected to colorimetric analysis at 500 nm. For the knockdown experiments, specific siRNAs were introduced to the cells using RNAiMAX reagent (Invitrogen) when they were ~50% confluent. The effective siRNA target sequences are listed in Supplementary Table S3 . Plasmids To construct pGL3-PGC-1α (PGC-1α/Luc), a luciferase reporter vector containing a mouse PGC-1 α gene promoter, the fragment (from −3,627 to +80) of this gene was PCR-amplified using primers containing Mlu I and Xho I sites at the 5′ and 3′ ends, respectively. The GAL4-DNA-binding domain-fused LSD1 expression vector, pcDNA3-GAL4-hLSD1wt, was generated by inserting the Eco RI- Not I fragment from pcDNA3-Flag-HA-hLSD1 (a gift from Dr Tadashi Baba) into the corresponding sites of pcDNA-GAL4mock. pcDNA3-GAL4-hLSD1mut, which expressed the FAD-binding motif-mutated LSD1, was prepared by site-directed mutagenesis. Two glycine-to-alanine mutations were introduced using the primer pair listed in Supplementary Table S4 . GAL4-binding motifs-containing reporter vector (pGL3-GALx5-SNRPN) was described previously [54] . Luciferase reporter assay Luciferase reporter analyses were performed using a dual-luciferase reporter assay system (Promega), according to the manufacturer's protocol. For PGC-1 α promoter analysis, the pGL3-PGC-1α reporter vector was co-transfected with the reference vector pRL-TK into 3T3-L1 cells, followed by 24-hour adipogenic induction before luciferase measurement. The siRNAs were introduced 24 h before the reporter transfection. For GAL4 reporter assay, pcDNA-GAL4 plasmids were co-transfected with the reporter plasmid pGL3-GALx5-SNRPN and pRL-TK into 293T or 3T3-L1 cells. After 48-h culture, the cells were collected for luciferase measurement. RFK siRNA was introduced 24 h before plasmid transfection, whereas lumiflavin was added to the culture 24 h before the measurement. Gene-expression analysis Total RNA from tissues and cells were extracted using Trizol reagents (Invitrogen). Complementary DNAs were produced using SuperScript III reverse transcriptase (Invitrogen). Quantitative RT–PCR was performed by the SYBR green method using Thunderbird reagents (Toyobo) and ABI 7500 Sequence Detector (Applied Biosciences). Primers used in this study are listed in Supplementary Table S4 . Microarray analysis Genome-wide expression analysis was performed using a GeneChip Mouse Genome Array 430 2 in combination with a GeneChip Hybridization, Wash and Stain Kit (Affymetrix). Microarray data were repeatedly confirmed at Takara Dragon Genomics Center (Ohtsu, Japan). siRNA-introduced and TC-treated 3T3-L1 cells were induced to differentiate for 24 h followed by RNA extraction and a quality check using a Bioanalyzer RNA 6000 Nano Assay (Agilent). Data annotation analysis was performed using GeneSpring GX software (Agilent). Gene set enrichment analysis was performed using GSEA ver. 2.0 software provided by the Broad Institute of MIT and Harvard ( http://www.broadinstitute.org/gsea/ ). The accession number of the microarray data in GEO is GSE18600 . Chromatin immunoprecipitation and co-IP In the ChIP experiments for detecting modified histones, cells were crosslinked with 1% formaldehyde [55] . Following the cell lysis, isolated nuclei were subjected to sonication for chromatin fragmentation. Chromatin fragments were incubated at 4 °C overnight with appropriate antibodies, followed by a pull-down assay using protein A/G-conjugated agarose beads. Purified DNAs were subjected to quantitative PCR (qPCR) using the primer sets listed in Supplementary Table S4 . To detect LSD1 enrichment on the genomic DNAs, we employed a protocol for detecting indirect associations between protein and DNA [56] . Briefly, enhanced crosslinking of chromatin using formaldehyde and protein-protein chemical crosslinker DTBP (dimethyl 3, 3′-dithiobispropionimidate 2HCl) (Sigma) was performed to increase the stability of protein-DNA complexes. Chromatin fragmentation was done by sonication in a regular RIPA buffer containing 0.1% SDS, followed by immunoprecipitation, as described above. For co-IP experiments, cells were lysed in IP buffer (50 mM Tris–HCl pH 8.0, 5 mM EDTA 150 mM NaCl, 0.5% NP-40, 0.5% Triton-X100) and incubated with specific antibodies followed by the pull-down with protein A-sepharose beads for subsequent western blot analyses. Generation of adenoviral vectors that express shRNA The 65-bp oligonucleotides containing specific shRNA for LSD1 (5′-GATCCCACAAGGAAAGCTAGAAGATTCAAGAGATCTTCTAGCTTTCCTTGTGTTTTTTACGCGTG-3′; the target sequence is underlined), BHC80 (5′-GATCCGTTCCAGATACAGCCATTGTTCAAGAGACAATGGCTGTATCTGGAACTTTTTTACGCGTG-3′) and control GL3 (5′-GATCCGATTTCGAGTCGTCTTAATTTCAAGAGAATTAAGACGACTCGAAATCTTTTTTACGCGTG-3′) (synthesized by TaKaRa Bio Company) were ligated to the BamHI and EcoRI sites of RNAi-Ready pSIREN-Shuttle Vector (Clontech Laboratories). and were subsequently sequenced for verification. The DNA fragment containing LSD1, BHC80 or GL3-specific shRNA downstream to the human U6 promoter was subcloned into adenoviral vector plasmid pAd.HM4, and was transfected to 293 cells. The generated replication-deficient adenoviral vector was propagated, purified and tittered, as described previously [57] , [58] . Expression of shRNA in isolated adipose tissues For ex vivo adipose tissue culture, epididymal WAT of mice was obtained, dissected into ~3-mm cubes and maintained in primary culture medium (DMEM/F12 (1:1) supplemented with 10% FBS, 100 μM ascorbic acid, 100 nM insulin and 200 pM 3, 3′, 5-triiodo L -thyronine). For adenovirus infection, three tissue blocks were placed into a single well of 48-well plate and exposed to adenovirus expressing either control or LSD1 shRNA at a MOI of 1.5×10 8 plaque-forming units (pfu) per well. Infections were repeated in triplicate wells for each virus. In vivo introduction of adenoviruses We used adenovirus transiently expressing LSD1 shRNAs in WAT in vivo , because LSD1-deficient mice and cells had severe defects [11] . For in vivo LSD1-knockdown experiments, adenoviruses were directly injected into the epididymal WAT of HFD-fed mice. Under anaesthesia, the outer coats of mice were dissected at the lower part of the abdomen. In obese mice, a portion of epididymal WAT was visible through the peritoneum, enabling targeted injection of adenoviruses. Adenoviruses expressing either control or LSD1 shRNAs were injected into the epididymal WAT on the right side of the abdomen at a MOI of 5×10 8 pfu per mouse. Four days after injection, tissues were collected for RNA analyses. Assessment of cellular metabolism For the determination of mitochondrial metabolism, 3T3-L1 cells were stained with fluorescence dye JC-1, followed by flow cytometric analysis [32] . Following trypsinization, cells were exposed to 5 μg ml −1 of JC-1 in the culture medium for 15 min at 37 °C and were suspended in PBS for fluorescence-activated cell sorting (FACS) analysis. Green and red fluorescent signals detected mitochondrial mass (FL1) and mitochondrial membrane potential (FL2), respectively, using a FACS Canto cytometer (Becton Dickinson). Cellular lipolytic activity was determined by measuring the concentration of free glycerol released into the culture medium during the 24-h culture, using an Adipolysis Assay Kit (Cayman Chemical). Cellular lactate content was measured using a Lactate Assay Kit II (BioVision), according to the manufacturer's instructions. Oxygen consumption was measured using a BD Oxygen Biosensor (BD Falcon), according to the manufacturer's instructions. For the assay, adipocytes were dispersed into single cells by Accumax reagent (Innovative Cell Technologies) and resuspended in the culture medium. Cell numbers were calculated for the normalization of the oxygen consumption values. Oxygen consumption rate (OCR) values were calculated as the fold-increase during a 30-min-measurement. Real-time measurement of OXPHOS activity Real-time monitoring of cellular OXPHOS activity was performed using XF24 Extracellular Flux Analyzer (Seahorse Bioscience), according to the manufacturer's instructions. siRNA-introduced 3T3-L1 cells were inoculated on the assay culture plate and allowed to differentiate for 24 h before the assay. Maximum OXPHOS capacity was determined as previously reported with some modifications [59] . In brief, during the real-time measurement, inhibitors of respiratory chain components were serially added to the culture. First, the complex V inhibitor, oligomycin (1 μg ml −1 ), was added followed by the addition of the respiratory uncoupler, carbonyl cyanide- p -trifluoromethoxyphenylhydrazone (FCCP) (1 μM), and then the complex I and III inhibitors, rotenone (100 nM) and antimycin A (10 μM). After each drug addition, the OCR was measured four times. The addition of FCCP accelerates oxygen consumption to a maximum level, whereas complex I inhibitors completely abolish the mitochondrial respiration. Thus, the difference in OCR between FCCP- and rotenone/antimycin-added states indicates the maximum OXPHOS capacity. Statistical analyses Data are presented as means±s.d. All statistical analyses were performed by a two-tailed Student's t -test, except in the microarray experiments, in which Pearson's χ 2 test was carried out. Accession codes: The microarray data have been deposited in the GEO database under accession code GSE18600 . How to cite this article: Hino, S. et al . FAD-dependent lysine-specific demethylase-1 regulates cellular energy expenditure. Nat. Commun. 3:758 doi: 10.1038/ncomms1755 (2012).